PDGFRβ signalling regulates local inflammation and synergizes with hypercholesterolaemia to promote atherosclerosis Platelet-derived growth factor (PDGF) is a mitogen and chemoattractant for vascular smooth muscle cells (VSMCs). However, the direct effects of PDGF receptor β (PDGFRβ) activation on VSMCs have not been studied in the context of atherosclerosis. Here we present a new mouse model of atherosclerosis with an activating mutation in PDGFRβ. Increased PDGFRβ signalling induces chemokine secretion and leads to leukocyte accumulation in the adventitia and media of the aorta. Furthermore, PDGFRβ D849V amplifies and accelerates atherosclerosis in hypercholesterolemic ApoE −/− or Ldlr −/− mice. Intriguingly, increased PDGFRβ signalling promotes advanced plaque formation at novel sites in the thoracic aorta and coronary arteries. However, deletion of the PDGFRβ-activated transcription factor STAT1 in VSMCs alleviates inflammation of the arterial wall and reduces plaque burden. These results demonstrate that PDGFRβ pathway activation has a profound effect on vascular disease and support the conclusion that inflammation in the outer arterial layers is a driving process for atherosclerosis. Atherosclerosis is a disease of the arteries that remains one of the leading causes of death and disability worldwide. It is characterized by the formation of fatty-fibrous plaques at specific arterial sites through a decade-long process driven by lipoprotein deposition in the vessel wall. This stimulus initiates a cascade of events including leukocyte recruitment and foam cell formation, vascular smooth muscle cell (VSMC) proliferation, changes in extracellular matrix, angiogenesis, calcification and cell death [1] , [2] , [3] . Most plaques are asymptomatic unless they obstruct blood flow. Other plaques are vulnerable to rupture, which can trigger thrombosis and a deadly risk of sudden heart attack or stroke. However, the interplay of these disease events is not fully understood and is still being explored mechanistically. Animal models have been invaluable for understanding disease mechanisms in atherosclerosis. The most widely used models are mice with hypercholesterolaemia caused by deficiency for apolipoprotein E ( ApoE −/− ) or low-density lipoprotein (LDL) receptor ( Ldlr −/− ). These animals develop atherosclerosis over several months compared with decades in humans. However, they do not form the types of advanced plaques that are clinically relevant in humans, nor do they typically develop coronary plaques or experience spontaneous death from heart attack or stroke [4] , [5] , [6] . Therefore, our understanding of advanced plaques is mostly based on descriptive findings from human autopsy studies. To develop a mechanistic understanding of advanced disease processes it is important to generate improved mouse models. Advanced atherosclerotic plaques develop a morphologically distinct fibrous cap composed of VSMCs that proliferate and migrate from the vessel wall into the plaque [7] , [8] , [9] . Platelet-derived growth factor (PDGF) was first purified over 30 years ago as a serum-derived factor that stimulates VSMC proliferation and migration [10] , [11] . PDGF is also a potent inducer of VSMC phenotype switching, or dedifferentiation, wherein VSMCs change from a mature, contractile phenotype to a proliferative, secretory phenotype [8] , [12] , [13] . PDGF signalling occurs via PDGF receptors (PDGFRs), which are prototypical of receptor tyrosine kinases. In the absence of PDGF ligand, PDGFR tyrosine kinase activity is inhibited by an autoinhibitory allosteric conformation; ligand binding alters the conformation to allow physiological signalling activity. PDGF signalling via PDGFRβ has been associated with vascular disease and is suspected to play a major role in VSMC migration and proliferation during atherosclerosis [14] , [15] . In ApoE −/− mice, blockade of the PDGF–PDGFRβ pathway with neutralizing antibodies or chemical inhibitors reduced VSMC involvement in atherosclerosis [16] , [17] . It seems likely that increased PDGF signalling would stimulate more VSMC involvement in atherosclerosis and potentially drive the formation of more aggressive atherosclerosis in mice. This approach has not been explored previously. Here we take advantage of knockin mice having a Cre-inducible D849V point mutation in the endogenous PDGFR β gene ( PDGFRβ D849V ) [18] , which we activate with a Sm22α-Cre driver to initiate signalling in VSMCs. The D849V mutation destabilizes the autoinhibited conformation of the receptor and thereby increases basal and ligand-mediated PDGFRβ signalling. We show that PDGF signalling increases chemokine signalling from VSMCs and causes inflammation of the aorta, in addition to causing VSMC phenotype switching and architectural changes in the muscle layer of the aorta. Using this model, we test the hypothesis that PDGF-driven changes in VSMC phenotype and function synergize with hypercholesterolaemia to promote the formation of advanced atherosclerotic plaques. Surprisingly, increased PDGF signalling not only promotes the formation of advanced plaque morphologies but it also enhances the initiation of new plaques at a plaque-resistant site, the thoracic aorta. Cells respond to PDGF signalling by phosphorylating transcription factors of the signal transducer and activator of transcription (STAT) family, and STAT1 in particular is known to regulate chemokine gene expression. Experiments with the kinase inhibitor Ruxolitinib (Rux) suggest that PDGFRβ phosphorylation of STAT1 requires the activity of Janus-activated kinase 1/2 (JAK1/2) tyrosine kinases. By deletion of a STAT1-floxed allele in VSMCs, we show that PDGF-driven chemokine signalling and inflammation are STAT1 dependent. Finally, in the context of PDGF-driven atherosclerosis, deletion of STAT1 from VSMCs reduces plaque formation, demonstrating that inflammation of the arterial media and adventitia are important mechanisms by which PDGF signalling promotes atherosclerosis. PDGF signalling induces chemokine production from VSMCs We previously showed that a Cre-inducible gain-of-function knockin mutation in PDGFRβ (PDGFRβ D849V ) induced chemokine mRNA expression in brain pericytes and caused inflammation of the central nervous system [18] . To characterize chemokine expression specifically in VSMCs of the aorta, which was not previously tested, we generated Sm22α-Cre;PDGFRβ +/D849V ( PDGFRβ Sm22D849V ) conditional mutant mice and Sm22α-Cre;PDGFRβ +/+ littermate controls (designated as Wt, Wild type) ( Fig. 1a ). We then established primary VSMC cultures from mutant and control aortas and examined the expression of chemokines that we previously identified by microarray. Using quantitative reverse transcription–PCR (qRT–PCR), we found upregulated mRNA levels for chemokines known to regulate monocyte (CCL2, CCL3, CCL5, CCL6, CCL7, CCL9, CCL12) and T-cell recruitment (CXCL9, CXCL10, CXCL11) ( Fig. 1b ). We also detected increased chemokine secretion in conditioned media from mutant VSMCs ( Fig. 1c ). Mouse plasma contains much lower levels of chemokines compared with conditioned media, but even with this limitation we detected increased levels of circulating CCL2 and CCL3 in the plasma of PDGFRβ Sm22D849V mice ( Fig. 1d ). Chemokine expression could be induced by treating control VSMCs with PDGF-BB ( Fig. 1e ). However, other known inflammatory signals, namely IL-1β, TNF-α, IFN-α, IFN-β and IFN-γ, were not upregulated in mutant VSMCs compared with controls (by qRT–PCR, data not shown). Thus, PDGFRβ signalling in VMSCs induces several chemokines, many of which are known to be involved in atherosclerosis [19] . 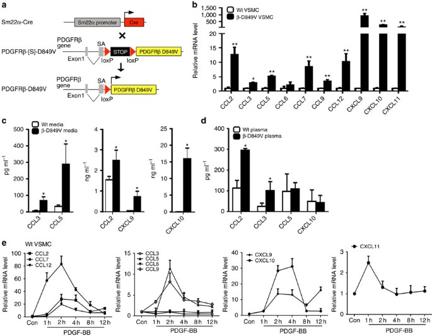Figure 1: PDGF signalling induces VSMCs to release chemokines. (a) Strategy for activating a conditionalPDGFRβD849Vallele in VSMCs. The conditionalPDGFRβD849Vallele consists of a loxP-flanked stop cassette preceding a full-length mouse PDGFRβ complementary DNA with a single amino acid substitution (D849V), which was targeted to thePdgfrβgene. When the conditional allele is present in Sm22α-Cre transgenic mice, the stop is removed in VSMCs and PDGFRβD849Vis expressed. SA, splice acceptor. (b) Fold change in chemokine mRNA levels in cultured VSMCs fromPDGFRβSm22D849V(β-D849V) mutant mice and Sm22α-Cre (Wt) control mice was determined by quantitative RT–PCR. Results are shown as fold increase in mutant over control,n=3 different VSMC isolates per genotype. (c) Quantification of chemokines secreted into the media of cultured VSMCs as determined by ELISA,n=3 different VSMC isolates per genotype. (d) Quantification of chemokines in plasma from mutant mice and control mice as determined by ELISA,n=3 mice per genotype. (e) Fold change in chemokine mRNA levels in cultured Wt VSMCs treated with 10 ng ml−1PDGF-BB ligand for the indicated times was determined by quantitative RT–PCR. Results are shown as fold increase in treated cells over untreated controls,n=3 different VSMC isolates. All data were assessed using Student’st-test and are present as mean±s.e.m. *P<0.05; **P<0.01. Figure 1: PDGF signalling induces VSMCs to release chemokines. ( a ) Strategy for activating a conditional PDGFRβ D849V allele in VSMCs. The conditional PDGFRβ D849V allele consists of a loxP-flanked stop cassette preceding a full-length mouse PDGFRβ complementary DNA with a single amino acid substitution (D849V), which was targeted to the Pdgfrβ gene. When the conditional allele is present in Sm22α-Cre transgenic mice, the stop is removed in VSMCs and PDGFRβ D849V is expressed. SA, splice acceptor. ( b ) Fold change in chemokine mRNA levels in cultured VSMCs from PDGFRβ Sm22D849V (β-D849V) mutant mice and Sm22α-Cre (Wt) control mice was determined by quantitative RT–PCR. Results are shown as fold increase in mutant over control, n =3 different VSMC isolates per genotype. ( c ) Quantification of chemokines secreted into the media of cultured VSMCs as determined by ELISA, n =3 different VSMC isolates per genotype. ( d ) Quantification of chemokines in plasma from mutant mice and control mice as determined by ELISA, n =3 mice per genotype. ( e ) Fold change in chemokine mRNA levels in cultured Wt VSMCs treated with 10 ng ml −1 PDGF-BB ligand for the indicated times was determined by quantitative RT–PCR. Results are shown as fold increase in treated cells over untreated controls, n =3 different VSMC isolates. All data were assessed using Student’s t -test and are present as mean±s.e.m. * P <0.05; ** P <0.01. Full size image PDGF signalling in VSMCs causes inflammation of the aorta Based on our finding of increased chemokine secretion by PDGFRβ Sm22D849V VSMCs, we sought to assess the resident leukocyte populations in the wall of the aorta. By flow-cytometric analysis of enzymatically digested control and mutant thoracic aortas, we found that mutants carried a sevenfold increase in the total number of CD45 + leucocytes ( Fig. 2a,b and Supplementary Fig. 1 ). The majority of the leucocytes were found in the adventitia, which is a normal site for small populations of leucocytes to reside in a non-atherosclerotic aorta ( Fig. 2c ) [20] , [21] , [22] . Histological analysis also provided evidence of abundant accumulated leucocytes in the mutant aorta adventitia and media ( Fig. 2d ). Further flow-cytometric analysis revealed increased numbers of leucocytes expressing CD3, CD19, CD11b, CD11c and NK1.1 in the mutant aortas ( Fig. 2e ). These data suggest that PDGF signalling in VSMCs induces signals, likely to be chemokines, which create an inflammatory milieu in the wall of the thoracic aorta. To investigate whether short-term pharmacological inhibition of PDGFRβ could reduce inflammation in the vessel wall, we treated PDGFRβ Sm22D849V mice with Crenolanib, a tyrosine kinase inhibitor specific for class III receptors. After 5 days of treatment, we found a decrease in the number of leucocytes in mutants that received the drug compared with untreated mutants ( Fig. 2f,g ). This suggests that continual PDGFRβ activation sustains inflammation. 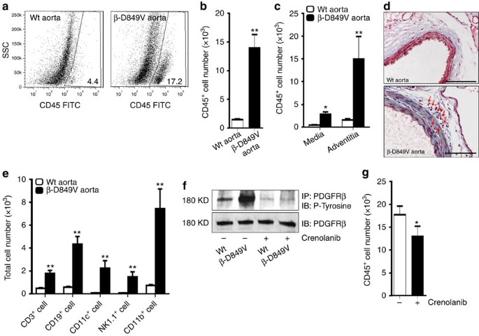Figure 2: PDGF signalling in VSMCs causes inflammation of the aorta. (a) Flow-cytometric analysis of cells in the aorta ofPDGFRβSm22D849V(β-D849V) mutant mice and Sm22α-Cre (Wt) control mice after enzymatic digestion. Numerical data indicate the percentage of CD45+leucocytes among the total cells analysed. Representative plots from three aortas of each genotype are shown. (b,c) Quantification of CD45+leucocytes in the whole aorta or the separated media and adventitia as measured by flow cytometry,n=3 mice per genotype for each type of analysis. (d) Distribution of leucocytes (red arrows) in the media and adventitia was determined by staining cross-sections of the thoracic aorta with Masson’s trichrome. Representative sections from three aortas of each genotype are shown. Scale bar, 100 μm. (e) Quantification of immune cell types in the aortic wall as measured by flow cytometry using fluorescent-conjugated antibodies: APC-CD3; APC.Cy7-CD19; PE-CD11c; PE.Cy7-NK1.1; PerCy5.5-Mac1,n=3 mice per genotype. (f) Phosphorylation of immunoprecipitated PDGFRβ from cultured VSMCs was determined by western blotting with anti-phosphotyrosine antibody. PDGFRβ-D849V tyrosine kinase activity was inhibited by treatment with the PDGFR inhibitor Crenolanib (400 ng ml−1) for 2 h prior to cell lysis. Representative blot from two experiments is shown. (g) Quantification of CD45+leukocytes in the whole aorta ofPDGFRβSm22D849Vmutant mice was measured by flow cytometry. Injecting mice with 15 mg kg−1Crenolanib for 5 consecutive days before sacrifice led to attenuation of CD45+leucocytes in the aortic wall,n=3 mice per treatment. All data were assessed using Student’st-test and are present as mean±s.e.m. *P<0.05; **P<0.01. Figure 2: PDGF signalling in VSMCs causes inflammation of the aorta. ( a ) Flow-cytometric analysis of cells in the aorta of PDGFRβ Sm22D849V (β-D849V) mutant mice and Sm22α-Cre (Wt) control mice after enzymatic digestion. Numerical data indicate the percentage of CD45 + leucocytes among the total cells analysed. Representative plots from three aortas of each genotype are shown. ( b , c ) Quantification of CD45 + leucocytes in the whole aorta or the separated media and adventitia as measured by flow cytometry, n =3 mice per genotype for each type of analysis. ( d ) Distribution of leucocytes (red arrows) in the media and adventitia was determined by staining cross-sections of the thoracic aorta with Masson’s trichrome. Representative sections from three aortas of each genotype are shown. Scale bar, 100 μm. ( e ) Quantification of immune cell types in the aortic wall as measured by flow cytometry using fluorescent-conjugated antibodies: APC-CD3; APC.Cy7-CD19; PE-CD11c; PE.Cy7-NK1.1; PerCy5.5-Mac1, n =3 mice per genotype. ( f ) Phosphorylation of immunoprecipitated PDGFRβ from cultured VSMCs was determined by western blotting with anti-phosphotyrosine antibody. PDGFRβ-D849V tyrosine kinase activity was inhibited by treatment with the PDGFR inhibitor Crenolanib (400 ng ml −1 ) for 2 h prior to cell lysis. Representative blot from two experiments is shown. ( g ) Quantification of CD45 + leukocytes in the whole aorta of PDGFRβ Sm22D849V mutant mice was measured by flow cytometry. Injecting mice with 15 mg kg −1 Crenolanib for 5 consecutive days before sacrifice led to attenuation of CD45 + leucocytes in the aortic wall, n =3 mice per treatment. All data were assessed using Student’s t -test and are present as mean±s.e.m. * P <0.05; ** P <0.01. Full size image Constitutive dedifferentiation of VSMCs As suggested previously [18] , PDGFRβ Sm22D849V mutant mice have constitutively dedifferentiated VSMCs and exhibit VSMC hyperplasia ( Fig. 3a ), decreased expression of contractile proteins SMMHC, SM22α and αSMA ( Fig. 3b ), and increased extracellular matrix production ( Fig. 3c,d ). Further analysis showed a cellular ultrastructure consistent with a phenotypic switch, where instead of contractile bundles there was an abundance of rough endoplasmic reticulum in mutant VMSCs ( Fig. 3e ). Due to VSMC hyperplasia and stiffening of the vessel wall, the thoracic aorta in PDGFRβ Sm22D849V mutants undergoes adaptive remodelling to become approximately twofold larger in diameter by 4 weeks of age, as shown previously [18] . We found no significant difference in blood pressure between adult mutants and controls (mutant: systolic 96.6±2.8/diastolic 73.3±5.8 mm Hg; control: systolic 108.3±8.3/diastolic 77.6±4.2 mm Hg; mean±s.e.m., n =6 mice per genotype). 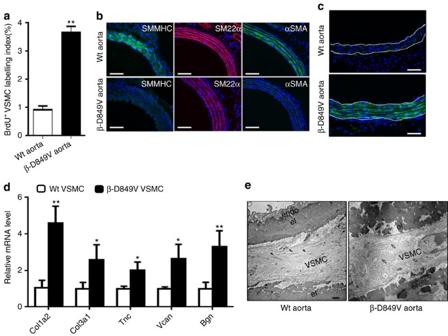Figure 3:PDGFRβSm22D849Vmutant mice have constitutively dedifferentiated VSMCs. (a) Proliferation of VSMCs in the thoracic aorta of 4-week-oldPDGFRβSm22D849V(β-D849V) mutant or Sm22α-Cre (Wt) control mice was measured by immunohistochemical detection of BrdU incorporation. Data represent the percentage of VSMCs that were BrdU+,n=3 aortas per genotype. (b) Mature VSMC marker expression in the cross-sectioned thoracic aorta of 4-week-old mice was determined by immunofluorescence, with DAPI as a nuclear counterstain. Representative images from three aortas of each genotype are shown. Scale bar, 50 μm. (c) Expression of a Collagen1a1-EGFP transgenic reporter in mutant or control mice was determined by epifluorescence with DAPI as a nuclear counterstain. The media is outlined. Representative images from three aortas of each genotype are shown. Scale bar, 50 μm. (d) Fold change in extracellular matrix protein mRNA levels in cultured VSMCs from mutant and control mice was determined by quantitative RT–PCR. Results are shown as fold increase in mutant over control,n=4 cell isolates per genotype. (e) VSMC ultrastructure in the thoracic aorta of 2-week-old mutant or control mice was determined by transmission electron microscopy. Black arrows identify VSMC contractile bundles in the control; open arrows identify rough endoplasmic reticulum in the mutant; endo, endothelium; el, elastic lamellae. Scale bar, 50 nm. All data were assessed using Student’st-test and are present as mean±s.e.m. *P<0.05; **P<0.01. Figure 3: PDGFRβ Sm22D849V mutant mice have constitutively dedifferentiated VSMCs. ( a ) Proliferation of VSMCs in the thoracic aorta of 4-week-old PDGFRβ Sm22D849V (β-D849V) mutant or Sm22α-Cre (Wt) control mice was measured by immunohistochemical detection of BrdU incorporation. Data represent the percentage of VSMCs that were BrdU + , n =3 aortas per genotype. ( b ) Mature VSMC marker expression in the cross-sectioned thoracic aorta of 4-week-old mice was determined by immunofluorescence, with DAPI as a nuclear counterstain. Representative images from three aortas of each genotype are shown. Scale bar, 50 μm. ( c ) Expression of a Collagen1a1-EGFP transgenic reporter in mutant or control mice was determined by epifluorescence with DAPI as a nuclear counterstain. The media is outlined. Representative images from three aortas of each genotype are shown. Scale bar, 50 μm. ( d ) Fold change in extracellular matrix protein mRNA levels in cultured VSMCs from mutant and control mice was determined by quantitative RT–PCR. Results are shown as fold increase in mutant over control, n =4 cell isolates per genotype. ( e ) VSMC ultrastructure in the thoracic aorta of 2-week-old mutant or control mice was determined by transmission electron microscopy. Black arrows identify VSMC contractile bundles in the control; open arrows identify rough endoplasmic reticulum in the mutant; endo, endothelium; el, elastic lamellae. Scale bar, 50 nm. All data were assessed using Student’s t -test and are present as mean±s.e.m. * P <0.05; ** P <0.01. Full size image PDGF signalling amplifies atherosclerosis Inflammation, VSMC dedifferentiation and aortic enlargement in PDGFRβ Sm22D849V mice provided clues that they might be more susceptible to atherosclerosis than normal mice. In particular, vascular inflammation is an early event in atherosclerosis, and VSMC dedifferentiation is characteristic of later disease. However, the most important risk factor for atherosclerosis is high cholesterol and PDGFRβ Sm22D849V mice had normal cholesterol and triglyceride levels compared with control counterparts ( Table 1 ). Accordingly, we did not detect atherosclerotic plaques up to 1 year of age whether the mutants were fed a normal chow or Western diet (WD). Therefore, to produce hypercholesterolaemia we backcrossed PDGFRβ Sm22D849V mice onto an ApoE -deficient genetic background to generate ApoE −/− ;Sm22α-Cre;PDGFRβ +/D849V ( ApoE,PDGFRβ Sm22D849V ) mutant mice and ApoE −/− ;Sm22α-Cre;PDGFRβ +/+ ( ApoE ) littermate controls. Thus, serum lipid profiles increased as expected ( Table 1 ). Table 1 Serum lipid profiles. Full size table After 16 weeks of WD, we assessed atherosclerotic plaque formation by two common methods: Oil red O staining for plaques on the luminal surface of flat-mounted aortas, and cross-sectional analysis of plaques in the aortic root. Both approaches revealed a dramatic increase in plaque formation in ApoE,PDGFRβ Sm22D849V mice. Flat-mounted ApoE aortas exhibited plaques in the aortic arch, the brachiocephalic artery and occasionally at branch points to the renal arteries, which are typical sites of plaque formation. In contrast, ApoE,PDGFRβ Sm22D849V aortas exhibited confluent plaques throughout the aortic tree, including the typically plaque-resistant thoracic aorta ( Fig. 4a ). Similarly, plaques in the aortic root were larger in the ApoE,PDGFRβ Sm22D849V mice and they exhibited an advanced morphology with well-defined fibrous caps overlying acellular necrotic cores ( Fig. 4b ). Necrotic core area was much larger and fibrous cap thickness was reduced in ApoE,PDGFRβ Sm22D849V aortic root plaques compared with ApoE ( Supplementary Fig. 2b,c ). ApoE,PDGFRβ Sm22D849V aortic root plaques were enriched for macrophages as a per cent of plaque area ( Supplementary Fig. 2a ). Gene expression analysis suggested that macrophages in ApoE,PDGFRβ Sm22D849V plaques were more of the M1 (pro-inflammatory) phenotype than M2, in comparison to ApoE ( Supplementary Fig. 3 ). 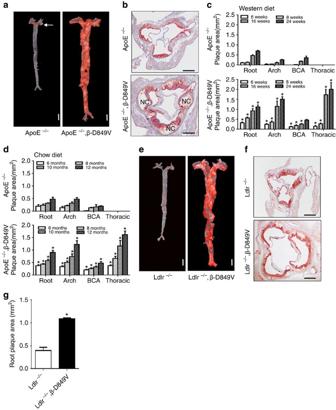Figure 4: PDGF signalling amplifies atherosclerosis in hypercholesterolemic mice. (a) Distribution of atherosclerotic plaques on the aortic lumen ofApoE,PDGFRβSm22D849V(ApoE−/−,β-D849V) mutants andApoE−/−controls after 16 weeks of WD was determined byen faceOil red O staining. Representative pictures of three aortas of each genotype are shown. Arrow indicates aortic arch plaques in theApoEcontrol. Scale bar, 5 mm. (b) Distribution of plaques in the aortic root after 16 weeks of WD was determined by staining sections with Oil red O. Representative pictures of three roots of each genotype are shown. NC, necrotic core. Scale bar, 500 μm. (c,d) Quantification of plaque cross-sectional area at the aortic root, aortic arch, brachiocephalic artery (BCA) and thoracic aorta in mice fed WD (c) or chow diet (d) for the indicated times,n=10 mice of each genotype per time point; *P<0.01 by Student’st-test for comparison between mutant and control at each time point. (e) Distribution of atherosclerotic plaques on the aortic lumen ofLdlr,PDGFRβSm22D849V(Ldlr−/−,β-D849V) mutants andLdlr−/−controls after 16 weeks of WD was determined byen faceOil red O staining. Representative pictures of three aortas of each genotype are shown. Scale bar, 5 mm. (f) Distribution of plaques in the aortic root after 16 weeks of WD was determined by staining sections with Oil red O. Representative pictures of six roots of each genotype are shown. Scale bar, 500 μm. (g) Quantification of plaque cross-sectional area in the aortic root,n=6 roots of each genotype; *P<0.01 by Student’st-test. All data represent mean±s.e.m. Figure 4: PDGF signalling amplifies atherosclerosis in hypercholesterolemic mice. ( a ) Distribution of atherosclerotic plaques on the aortic lumen of ApoE,PDGFRβ Sm22D849V (ApoE −/− ,β-D849V) mutants and ApoE −/− controls after 16 weeks of WD was determined by en face Oil red O staining. Representative pictures of three aortas of each genotype are shown. Arrow indicates aortic arch plaques in the ApoE control. Scale bar, 5 mm. ( b ) Distribution of plaques in the aortic root after 16 weeks of WD was determined by staining sections with Oil red O. Representative pictures of three roots of each genotype are shown. NC, necrotic core. Scale bar, 500 μm. ( c , d ) Quantification of plaque cross-sectional area at the aortic root, aortic arch, brachiocephalic artery (BCA) and thoracic aorta in mice fed WD ( c ) or chow diet ( d ) for the indicated times, n =10 mice of each genotype per time point; * P <0.01 by Student’s t -test for comparison between mutant and control at each time point. ( e ) Distribution of atherosclerotic plaques on the aortic lumen of Ldlr,PDGFRβ Sm22D849V (Ldlr −/− ,β-D849V) mutants and Ldlr −/− controls after 16 weeks of WD was determined by en face Oil red O staining. Representative pictures of three aortas of each genotype are shown. Scale bar, 5 mm. ( f ) Distribution of plaques in the aortic root after 16 weeks of WD was determined by staining sections with Oil red O. Representative pictures of six roots of each genotype are shown. Scale bar, 500 μm. ( g ) Quantification of plaque cross-sectional area in the aortic root, n =6 roots of each genotype; * P <0.01 by Student’s t -test. All data represent mean±s.e.m. Full size image To carefully track plaque progression over time, we quantified cross-sectional plaque area after 6, 8, 16 and 24 weeks of WD, measuring plaques in the aortic root, aortic arch, brachiocephalic artery and thoracic aorta ( Fig. 4c ). At all time points and all sites examined, plaques were significantly larger in ApoE,PDGFRβ Sm22D849V aortas. We also performed quantification of cross-sectional plaque area in a cohort of mice with chow diet feeding, where moderate hypercholesterolaemia results in slower plaque development. We examined time points between 6 and 12 months of age, and found that ApoE,PDGFRβ Sm22D849V aortas still developed distinctive plaques in the thoracic aorta and larger plaques at other sites compared with ApoE controls ( Fig. 4d ). We wanted to ensure that the synergistic effect of PDGF signalling and hypercholesterolaemia was not specific to the ApoE mutant. Therefore, we crossed PDGFRβ Sm22D849V mice with mice deficient for LDLR, which also causes hypercholesterolaemia. We compared Ldlr and Ldlr,PDGFRβ Sm22D849V mutants after 16 weeks of WD feeding and again found a striking increase in atherosclerotic plaque area in Ldlr,PDGFRβ Sm22D849V aortas ( Fig. 4e,f ). This finding is important because ApoE itself can influence PDGFRβ activity by interacting with LDL receptor-related protein-1 (LRP1) to attenuate PDGFRβ function [23] , [24] . The finding that PDGFRβ D849V synergizes with Ldlr argues that the effects shown here are not attributable to lack of inhibition from the ApoE–LRP1 complex. Taken together, the results from ApoE/WD, ApoE/chow and Ldlr/WD studies clearly demonstrate that increased PDGF signalling in VSMCs strongly amplifies atherosclerosis under a variety of hypercholesterolemic conditions. Plaque progression to fibroatheroma and haemorrhage We performed careful morphological assessment of the thoracic aorta plaques in ApoE,PDGFRβ Sm22D849V mice because of their striking size and unusual location. At 6 weeks of WD, the plaques initiated as accumulations of foam cell macrophages within the intima ( Fig. 5a , Supplementary Fig. 4 ). By 8 weeks of WD, smooth muscle cells were seen invading the foam cell-rich plaques and fibrous cap structures began to form at this time ( Fig. 5b , black arrows). By 16 and 24 weeks of WD, the plaques had reached a fibrous cap atheroma stage [4] , exhibiting well-formed collagen-rich fibrous caps and large necrotic cores ( Fig. 5c–e ). An additional feature seen at 16 weeks WD and later was areas of haemorrhage within advanced fibroatheroma plaques (seen in 7–10 mutants, Fig. 5f ). Cross-sectioning through such areas showed that haemorrhages were contained within the plaque without evidence of a ruptured fibrous cap ( Fig. 5g ). Iron deposition at haemorrhage sites was evident by Prussian blue stain ( Fig. 5h ). In advanced human atherosclerosis, neovascularization of plaques is associated with increased inflammation, intraplaque haemorrhage and increasing plaque vulnerability [25] , [26] . Accordingly, we observed PECAM + microvessels in advanced plaques of ApoE,PDGFRβ Sm22D849V mice ( Fig. 5i ). Together, these data demonstrate that ApoE,PDGFRβ Sm22D849V mice readily develop plaques with advanced morphologies much like those seen in humans. Fibroatheromas with these features are extremely rare (or nonexistent) in standard ApoE - and Ldlr -deficient mouse models. 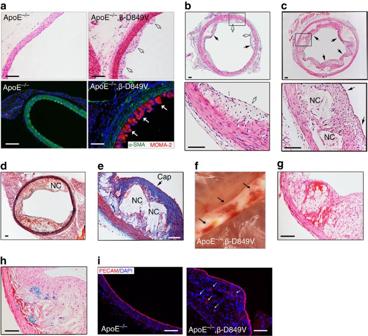Figure 5: Plaque initiation, progression to fibroatheroma and intraplaque haemorrhage. (a) Plaque initiation in the thoracic aorta ofApoE,PDGFRβSm22D849V(ApoE−/−,β-D849V) mutant andApoE−/−control mice after 6 weeks of WD was assessed by staining cross-sections of the aorta with haematoxylin and eosin (top panels) or with fluorescent antibodies to identify VSMCs (αSMA, green) and macrophage foam cells (MOMA-2, red). Representative pictures of three aortas of each genotype are shown. Only the mutant has subendothelial foam cell plaques in the thoracic aorta (white arrows). Scale bar, 100 μm. (b,c) Histological analysis of plaque progression in the thoracic aorta ofApoE,PDGFRβSm22D849Vmice after 8 weeks (b) or 24 weeks (c) of WD. Shown are low magnification pictures (top), and high magnification pictures of the boxed areas (bottom), which are representative of at least six mutant aortas analysed per time point. White arrows indicate foam cells, black arrows indicate fibrous caps, NC=necrotic core. Scale bar, 100 μm. (d,e) Histological analysis of advanced plaques inApoE,PDGFRβSm22D849Vmice after 16 or 24 weeks of WD. Sections were stained with (d) Movat’s pentachrome (16 weeks WD) or (e) Masson’s trichrome (24 weeks WD). Scale bar, 125 μm. (f) Digital photograph of three sites of haemorrhage (arrows) in theApoE,PDGFRβSm22D849Vthoracic aortain situafter 16 weeks of WD. Before photography, the mouse was perfused through the heart and the aorta was cleared of adipose tissue. (g,h) Histological analysis of intraplaque ruptures was performed with (g) haematoxylin and eosin or (h) Prussian blue and nuclear fast red to demonstrate intraplaque haemorrhage with no evidence of fibrous cap rupture. Scale bar, 100 μm. (i) Immunofluorescent analysis of endothelial cells in mutant andApoEcontrol thoracic aortas after 16 weeks of WD. Representative images of PECAM staining are shown. Arrows indicate neovessels in the mutant plaque. Scale bar, 100 μm. Figure 5: Plaque initiation, progression to fibroatheroma and intraplaque haemorrhage. ( a ) Plaque initiation in the thoracic aorta of ApoE,PDGFRβ Sm22D849V (ApoE −/− ,β-D849V) mutant and ApoE −/− control mice after 6 weeks of WD was assessed by staining cross-sections of the aorta with haematoxylin and eosin (top panels) or with fluorescent antibodies to identify VSMCs (αSMA, green) and macrophage foam cells (MOMA-2, red). Representative pictures of three aortas of each genotype are shown. Only the mutant has subendothelial foam cell plaques in the thoracic aorta (white arrows). Scale bar, 100 μm. ( b , c ) Histological analysis of plaque progression in the thoracic aorta of ApoE,PDGFRβ Sm22D849V mice after 8 weeks ( b ) or 24 weeks ( c ) of WD. Shown are low magnification pictures (top), and high magnification pictures of the boxed areas (bottom), which are representative of at least six mutant aortas analysed per time point. White arrows indicate foam cells, black arrows indicate fibrous caps, NC=necrotic core. Scale bar, 100 μm. ( d , e ) Histological analysis of advanced plaques in ApoE,PDGFRβ Sm22D849V mice after 16 or 24 weeks of WD. Sections were stained with ( d ) Movat’s pentachrome (16 weeks WD) or ( e ) Masson’s trichrome (24 weeks WD). Scale bar, 125 μm. ( f ) Digital photograph of three sites of haemorrhage (arrows) in the ApoE,PDGFRβ Sm22D849V thoracic aorta in situ after 16 weeks of WD. Before photography, the mouse was perfused through the heart and the aorta was cleared of adipose tissue. ( g , h ) Histological analysis of intraplaque ruptures was performed with ( g ) haematoxylin and eosin or ( h ) Prussian blue and nuclear fast red to demonstrate intraplaque haemorrhage with no evidence of fibrous cap rupture. Scale bar, 100 μm. ( i ) Immunofluorescent analysis of endothelial cells in mutant and ApoE control thoracic aortas after 16 weeks of WD. Representative images of PECAM staining are shown. Arrows indicate neovessels in the mutant plaque. Scale bar, 100 μm. Full size image Coronary atherosclerosis Coronary artery plaques are not typical in ApoE single mutant mice unless they are fed a WD for 10 months [27] , [28] . We observed coronary atherosclerosis in some of the PDGFRβ D849V cohorts. This was observed in 70% (7 of 10) of ApoE,PDGFRβ Sm22D849V mice that were fed a chow diet for 10–12 months ( Fig. 6a,b ) and in 71% (5 of 7) of Ldlr,PDGFRβ Sm22D849V mice that were fed WD for 16 weeks ( Fig. 6c,d ). Some of these plaques appeared to be fibroatheromas ( Fig. 6b ). Sudden deaths occurred in some ApoE,PDGFRβ Sm22D849V mice as early as 12 weeks of WD, and 50% died by 19 weeks of WD ( n =26) ( Supplementary Fig. 5 ). It is possible that coronary plaques contributed to the reduced viability of WD-fed mutants, but this needs to be investigated further in a study specifically designed to identify causes of death. 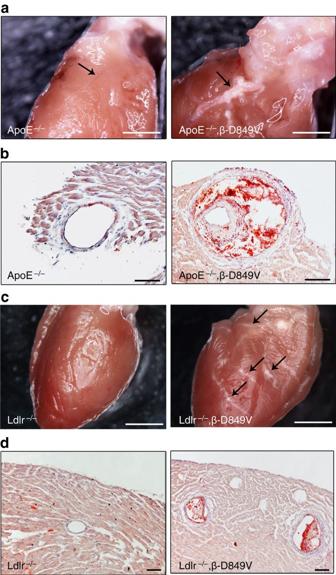Figure 6: Coronary atherosclerosis. (a) Coronary artery plaques appear inApoE,PDGFRβSm22D849Vmice after 10 months of chow diet but notApoEcontrol mice. Arrow indicates the left coronary artery. Pictures are representative of coronary plaques in 7 out of 10 mutants after >10 months of chow diet. (b) Cross-sections through the left coronary artery were stained with Oil red O and haematoxylin. Scale bar, 100 μm. (c) Coronary artery plaques inLdlr,PDGFRβSm22D849Vmice after 16 weeks of WD, but notLdlrcontrol mice. Arrows identify plaques in multiple arteries on the left anterior surface of the heart. Pictures are representative of plaques in five out of seven mutants after >16 weeks of WD. (d) Cross-sections through the heart were stained with Oil red O and haematoxylin. Scale bars, 1 mm (a), 200 μm (b,d), 2 mm (c). Figure 6: Coronary atherosclerosis. ( a ) Coronary artery plaques appear in ApoE,PDGFRβ Sm22D849V mice after 10 months of chow diet but not ApoE control mice. Arrow indicates the left coronary artery. Pictures are representative of coronary plaques in 7 out of 10 mutants after >10 months of chow diet. ( b ) Cross-sections through the left coronary artery were stained with Oil red O and haematoxylin. Scale bar, 100 μm. ( c ) Coronary artery plaques in Ldlr,PDGFRβ Sm22D849V mice after 16 weeks of WD, but not Ldlr control mice. Arrows identify plaques in multiple arteries on the left anterior surface of the heart. Pictures are representative of plaques in five out of seven mutants after >16 weeks of WD. ( d ) Cross-sections through the heart were stained with Oil red O and haematoxylin. Scale bars, 1 mm ( a ), 200 μm ( b , d ), 2 mm ( c ). Full size image PDGF signalling activates STAT1 in VSMCs The striking amplification of atherosclerosis raised mechanistic questions about which PDGF-regulated processes actually drive the atherosclerotic phenotype and which processes are bystanders. Clearly, inflammation is seen throughout atherogenesis. On the other hand, VSMC hyperplasia, phenotype switching and increased ECM synthesis seemed important for helping early plaques to progress to the fibroatheroma morphology. Therefore, we hypothesized that PDGF-induced chemokine secretion and inflammation of the vessel wall (see Figs 1 and 2 ) were the processes driving plaque initiation. PDGFRβ regulates several downstream signalling cascades including Ras/MAP kinase, PI3 kinase/AKT, PLCγ/PKC and STATs. We chose to focus on STAT1 as a potential mediator of pro-inflammatory PDGFRβ signalling because this transcription factor is a direct activator chemokine gene expression in the context of interferon (IFN) signalling [29] . First, PDGFRβ +/+ (Wt) control VSMCs were incubated with or without IFN-γ and STAT1 phosphorylation was assessed. IFN-γ was required for STAT1 phosphorylation in control VSMCs, but STAT1 was constitutively phosphorylated in PDGFRβ Sm22D849V cells ( Fig. 7a ). This was specific to STAT1, as STAT3 and STAT5 were not phosphorylated in mutant cells. Treatment of control VSMCs with PDGF resulted in STAT1 phosphorylation ( Fig. 7b ), and treatment of PDGFRβ Sm22D849V cells with the PDGFR inhibitor AG-1295 abolished STAT1 phosphorylation ( Fig. 7c,d ), indicating that constitutive STAT1 phosphorylation depends on PDGF pathway activity. AG-1295 had no effect on STAT1 phosphorylation in response to IFN-γ treatment ( Fig. 7e,f , fourth lane), indicating that PDGFRβ is not required for this response. The constitutively phosphorylated STAT1 in PDGFRβ Sm22D849V VSMCs could be further phosphorylated by the addition of exogenous IFN-γ ( Fig. 7e,f , seventh lane), suggesting that PDGFRβ Sm22D849V VSMCs remain capable of sensing IFN. However, as discussed previously, we did not detect increased IFN (IFN-α, -β or -γ) mRNA expression in PDGFRβ Sm22D849V VSMCs compared with control cells, consistent with the model that PDGFRβ signalling is responsible for the phosphorylation of STAT1. 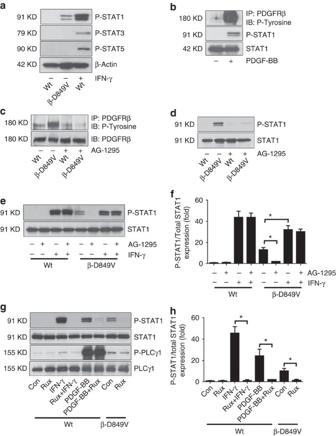Figure 7: PDGF signalling activates STAT1 in VSMCs. (a) Tyrosine phosphorylation of STAT1, STAT3 and STAT5 in cultured VSMCs fromPDGFRβSm22D849V(β-D849V) mutant and Sm22α-Cre (Wt) control mice was determined by western blot. As a positive control, VSMCs were treated with 10 ng ml−1mouse IFN-γ for 30 min. (b) Phosphorylation of PDGFRβ and STAT1 in control VSMCs after serum starvation and treatment with 10 ng ml−1PDGF-BB for 10 min was determined by western blot. PDGFRβ was immunoprecipitated from cell lysate and then phosphorylation was detected with anti-phosphotyrosine antibody. Phospho-STAT1 was detected in cell lysate with p-Y701 antibody. (c,d) PDGFRβ and STAT1 phosphorylation inPDGFRβSm22D849Vmutant and control VSMCs were analysed by western blotting after 16 h treatment with the PDGFR inhibitor 10 μM AG-1295. (e) STAT1 phosphorylation inPDGFRβSm22D849Vmutant and control VSMCs were analysed by western blotting after 16 h treatment with 10 μM AG-1295 followed by vehicle or 10 ng ml−1mouse IFN-γ for 30 min. (f) Quantification of western blots ineby densitometry shown as fold change over untreated Wt (lane 1). (g) STAT1 and PLCγ1 phosphorylation inPDGFRβSm22D849Vmutant and control VSMCs were analysed by western blotting after 16 h treatment with the JAK1/JAK2 inhibitor Ruxolitinib (10 μM) followed by 10 ng ml−1mouse IFN-γ for 30 min or 10 ng ml−1PDGF-BB for 10 min. (h) Quantification of western blots ingby densitometry shown as fold change over untreated Wt (lane 1). All data represent mean±s.e.m. All experiments were performed at least three times; *P<0.01 by Student’st-test. Figure 7: PDGF signalling activates STAT1 in VSMCs. ( a ) Tyrosine phosphorylation of STAT1, STAT3 and STAT5 in cultured VSMCs from PDGFRβ Sm22D849V (β-D849V) mutant and Sm22α-Cre (Wt) control mice was determined by western blot. As a positive control, VSMCs were treated with 10 ng ml −1 mouse IFN-γ for 30 min. ( b ) Phosphorylation of PDGFRβ and STAT1 in control VSMCs after serum starvation and treatment with 10 ng ml −1 PDGF-BB for 10 min was determined by western blot. PDGFRβ was immunoprecipitated from cell lysate and then phosphorylation was detected with anti-phosphotyrosine antibody. Phospho-STAT1 was detected in cell lysate with p-Y701 antibody. ( c , d ) PDGFRβ and STAT1 phosphorylation in PDGFRβ Sm22D849V mutant and control VSMCs were analysed by western blotting after 16 h treatment with the PDGFR inhibitor 10 μM AG-1295. ( e ) STAT1 phosphorylation in PDGFRβ Sm22D849V mutant and control VSMCs were analysed by western blotting after 16 h treatment with 10 μM AG-1295 followed by vehicle or 10 ng ml −1 mouse IFN-γ for 30 min. ( f ) Quantification of western blots in e by densitometry shown as fold change over untreated Wt (lane 1). ( g ) STAT1 and PLCγ1 phosphorylation in PDGFRβ Sm22D849V mutant and control VSMCs were analysed by western blotting after 16 h treatment with the JAK1/JAK2 inhibitor Ruxolitinib (10 μM) followed by 10 ng ml −1 mouse IFN-γ for 30 min or 10 ng ml −1 PDGF-BB for 10 min. ( h ) Quantification of western blots in g by densitometry shown as fold change over untreated Wt (lane 1). All data represent mean±s.e.m. All experiments were performed at least three times; * P <0.01 by Student’s t -test. Full size image In the IFN-γ signalling cascade, activated IFN receptors recruit JAK1 and -2, which are cytoplasmic tyrosine kinases that subsequently phosphorylate STAT1. Previous studies found that PDGFRβ associates with and phosphorylates JAK1, JAK2 and the related kinase Tyk2, but suggested that, unlike the IFN pathway, JAKs may be dispensable for PDGFRβ-induced STAT1 activation [30] , [31] . To explore this question in VSMCs, we treated control or mutant cells and the JAK1/2-selective inhibitor Rux. As expected, pretreatment of VSMCs with Rux blocked STAT1 phosphorylation in response to IFN-γ ( Fig. 7g,h , fourth lane). Interestingly, Rux also blocked STAT1 phosphorylation in control VSMCs treated with PDGF-BB, and in unstimulated PDGFRβ Sm22D849V VSMCs ( Fig. 7g,h , sixth and eighth lanes). This points to the conclusion that JAK1 and/or JAK2 are required for STAT1 phosphorylation in the PDGF signalling pathway. As a control, Rux had no effect on PDGFRβ-induced PLCγ1 phosphorylation, indicating that Rux does not impair PDGFRβ tyrosine kinase activity. STAT1 regulates chemokine production and inflammation We tested whether STAT1 could regulate chemokine expression using short interfering RNA (siRNA) knockdown and genetic approaches. Transfection of PDGFRβ Sm22D849V VSMCs with STAT1–siRNA significantly reduced total and phospho-STAT1 protein levels ( Fig. 8a ). qRT–PCR of PDGFRβ Sm22D849V VSMCs transfected with STAT1–siRNA showed reduced mRNA expression for 7 out of 10 chemokines compared with control siRNA ( Fig. 8b ). Next, we obtained STAT1 flox/flox mice [32] and bred them with PDGFRβ Sm22D849V mutants. Deletion of STAT1 protein from VSMCs was confirmed by western blot ( Fig. 8c ). We then compared chemokine expression in VSMCs from Wt, STAT1 Sm22CKO (STAT1-cKO) single mutant, PDGFRβ Sm22D849V (β-D849V) single mutant and STAT1 Sm22CKO PDGFRβ Sm22D849V (β-D849V,STAT1-cKO) double-mutant mice. In agreement with the siRNA knockdown, STAT1 Sm22cKO PDGFRβ Sm22D849V cells had significantly reduced expression of CCL2, CCL5, CCL7, CCL12, CXCL9, CXCL10 and CXCL11 compared with PDGFRβ Sm22D849V cells ( Fig. 8d ). Therefore, the PDGF signalling pathway regulates chemokine expression by a STAT1-dependent mechanism. We further investigated if STAT1 deletion could modify PDGFRβ-driven leukocyte accumulation in the aortic wall. We performed flow cytometry on thoracic aortas ( ApoE +/+ ) and found that CD45 + leukocyte accumulation was reduced to almost wild-type levels in STAT1 Sm22cKO PDGFRβ Sm22D849V aortas ( Fig. 8e , compare with Fig. 2b ). Interestingly, while STAT1 deletion prevented inflammation, downregulation of VSMC differentiation markers still occurred ( Fig. 8f , compare with Fig. 3b ) and aortic dilation was still observed. Thus, STAT1 regulates VSMC chemokine production and aortic inflammation downstream of PDGFRβ but it is not required for VSMC dedifferentiation. 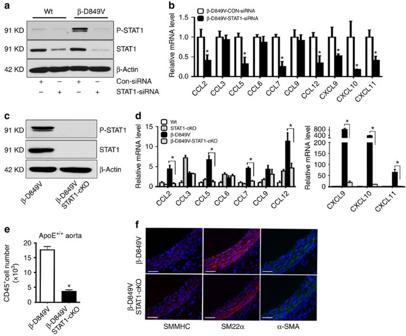Figure 8: STAT1 regulates chemokines and inflammation inPDGFRβSm22D849Vmice. (a) Expression of total STAT1 and STAT1 p-Y701 inPDGFRβSm22D849V(β-D849V) mutant and Sm22α-Cre (Wt) control VSMCs after transfection with control or STAT1-blocking siRNA was analysed by western blotting. (b) Fold change in chemokine mRNA levels in cultured VSMCs from mutant mice was determined by quantitative RT–PCR. Results are shown as fold change in STAT1 siRNA compared with control siRNA,n=4 transfections per siRNA. (c) Expression of total STAT1 and p-Y701 STAT1 inPDGFRβSm22D849V(β-D849V) single mutant andSTAT1Sm22CKOPDGFRβSm22D849V(β-D849V,STAT1-cKO) double-mutant VSMCs was analysed by western blotting. (d) Fold change in chemokine mRNA levels in Wt,STAT1Sm22CKO(STAT1-cKO),PDGFRβSm22D849V(β-D849V) single mutant andSTAT1Sm22CKOPDGFRβSm22D849V(β-D849V,STAT1-cKO) double-mutant VSMCs was determined by quantitative RT–PCR. Results are shown as fold change compared with Wt,n=3 different VSMC isolates per genotype. (e) Quantification of CD45+leucocytes in the whole aorta of single mutant and double-mutant mice (allApoE+/+) as measured by flow cytometry,n=3 mice per genotype. (f) Mature VSMC marker expression in the cross-sectioned thoracic aorta of 8-week-old mice was determined by immunofluorescence, with DAPI as a nuclear counterstain. Representative images from three aortas of each genotype are shown. Scale bar, 50 μm. All data were assessed using Student’st-test and are present as mean±s.e.m. *P<0.01. Figure 8: STAT1 regulates chemokines and inflammation in PDGFRβ Sm22D849V mice. ( a ) Expression of total STAT1 and STAT1 p-Y701 in PDGFRβ Sm22D849V (β-D849V) mutant and Sm22α-Cre (Wt) control VSMCs after transfection with control or STAT1-blocking siRNA was analysed by western blotting. ( b ) Fold change in chemokine mRNA levels in cultured VSMCs from mutant mice was determined by quantitative RT–PCR. Results are shown as fold change in STAT1 siRNA compared with control siRNA, n =4 transfections per siRNA. ( c ) Expression of total STAT1 and p-Y701 STAT1 in PDGFRβ Sm22D849V (β-D849V) single mutant and STAT1 Sm22CKO PDGFRβ Sm22D849V (β-D849V,STAT1-cKO) double-mutant VSMCs was analysed by western blotting. ( d ) Fold change in chemokine mRNA levels in Wt, STAT1 Sm22CKO (STAT1-cKO), PDGFRβ Sm22D849V (β-D849V) single mutant and STAT1 Sm22CKO PDGFRβ Sm22D849V (β-D849V,STAT1-cKO) double-mutant VSMCs was determined by quantitative RT–PCR. Results are shown as fold change compared with Wt, n =3 different VSMC isolates per genotype. ( e ) Quantification of CD45 + leucocytes in the whole aorta of single mutant and double-mutant mice (all ApoE +/+ ) as measured by flow cytometry, n =3 mice per genotype. ( f ) Mature VSMC marker expression in the cross-sectioned thoracic aorta of 8-week-old mice was determined by immunofluorescence, with DAPI as a nuclear counterstain. Representative images from three aortas of each genotype are shown. Scale bar, 50 μm. All data were assessed using Student’s t -test and are present as mean±s.e.m. * P <0.01. Full size image PDGF/STAT1-regulated inflammation amplifies atherosclerosis PDGFRβ Sm22D849V aortas exhibit inflammation and dedifferentiated VSMCs, and deletion of STAT1 in VSMCs reduces inflammation but does not affect the VSMC phenotype ( Fig. 8 ). This suggested that STAT1 deletion in ApoE,PDGFRβ Sm22D849V mice would be an approach to evaluate the importance of inflammation versus VSMC dedifferentiation as pro-atherosclerotic mechanisms. To test this, we generated ApoE,PDGFRβ Sm22D849V single conditional mutants with hypercholesterolaemia and ApoE −/− ;STAT1 flox/flox ;Sm22α-Cre;PDGFRβ +/D849V ( ApoE,STAT1 Sm22cKO PDGFRβ Sm22D849V ) double conditional mutants with hypercholesterolaemia. After feeding WD for 12 weeks, we screened for atherosclerosis. Compared with ApoE,PDGFRβ Sm22D849V mutants, a much smaller area of the aorta was covered by plaques in ApoE,STAT1 Sm22cKO PDGFRβ Sm22D849V mutants that were lacking STAT1 in VSMCs ( Fig. 9a,b ). Moreover, plaques in the aortic root of the double mutants were significantly smaller than those of the single mutants ( Fig. 9c,d ), appearing similar to the size of plaques in ApoE −/− aortic roots at 8–16 weeks of WD ( Fig. 4c ). Next, we examined plaque composition in the thoracic aorta. After 12 weeks of WD the less abundant plaques in ApoE,STAT1 Sm22cKO PDGFRβ Sm22D849V mutants were clearly less advanced with poorly developed fibrous caps and small necrotic cores compared with ApoE,PDGFRβ Sm22D849V mutants ( Fig. 9e ). Therefore, PDGFRβ-STAT1 signalling in VMSCs creates an inflammatory milieu in the aortic adventitia and media that strongly predisposes arteries to form atherosclerotic plaques in synergy with hypercholesterolaemia. 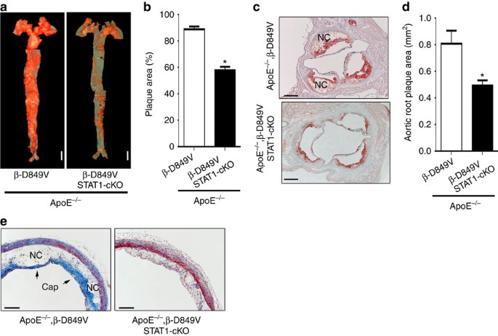Figure 9: PDGF/STAT1-regulated inflammation amplifies atherosclerosis. (a) Distribution of atherosclerotic plaques on the aortic lumen ofApoE,PDGFRβSm22D849Vmutants andApoE,STAT1Sm22CKOPDGFRβSm22D849Vdouble mutants after 12 weeks of WD was determined byen faceOil red O staining. Representative pictures of six aortas of each genotype are shown. Scale bar, 5 mm. (b) Quantification of plaque area as a percentage of total surface area of the aorta,n=6 aortas per genotype. (c) Distribution of plaques in the aortic root after 12 weeks of WD was determined by staining sections with Oil red O. Representative pictures of six roots of each genotype are shown. NC, necrotic core. Scale bar, 500 μm. (d) Quantification of plaque cross-sectional area in the aortic root,n=6 roots per genotype. (e) Histological analysis of plaque morphology in the thoracic aorta after 12 weeks of WD was determined by trichrome staining. Arrows indicate blue collagen staining in the fibrous cap. Scale bar, 250 μm. Representative pictures of three aortas of each genotype are shown. All data represent mean±s.e.m. *P<0.01 by Student’st-test. Figure 9: PDGF/STAT1-regulated inflammation amplifies atherosclerosis. ( a ) Distribution of atherosclerotic plaques on the aortic lumen of ApoE,PDGFRβ Sm22D849V mutants and ApoE,STAT1 Sm22CKO PDGFRβ Sm22D849V double mutants after 12 weeks of WD was determined by en face Oil red O staining. Representative pictures of six aortas of each genotype are shown. Scale bar, 5 mm. ( b ) Quantification of plaque area as a percentage of total surface area of the aorta, n =6 aortas per genotype. ( c ) Distribution of plaques in the aortic root after 12 weeks of WD was determined by staining sections with Oil red O. Representative pictures of six roots of each genotype are shown. NC, necrotic core. Scale bar, 500 μm. ( d ) Quantification of plaque cross-sectional area in the aortic root, n =6 roots per genotype. ( e ) Histological analysis of plaque morphology in the thoracic aorta after 12 weeks of WD was determined by trichrome staining. Arrows indicate blue collagen staining in the fibrous cap. Scale bar, 250 μm. Representative pictures of three aortas of each genotype are shown. All data represent mean±s.e.m. * P <0.01 by Student’s t -test. Full size image The mechanisms that control the initiation and progression of atherosclerosis are incompletely understood. In this study, we investigated the effects of increased PDGFRβ signalling on atherosclerosis. We first showed that conditional activation of PDGFRβ induced the expression of chemokines in VSMCs and caused inflammation of the aortic media and adventitia in PDGFRβ Sm22D849V mutant mice. Taken together with VSMC dedifferentiation, hyperplasia and increased ECM synthesis, these phenotypes suggested that the activating mutation in PDGFRβ would be pro-atherogenic. Analysis of ApoE,PDGFRβ Sm22D849V mice provided clear evidence that PDGF signalling strongly amplified hypercholesterolaemia-induced atherosclerosis. Intriguingly, increased PDGF signalling expanded the sites of plaque initiation, allowing atherosclerosis to occur in the thoracic aorta and coronary arteries that are typically free of plaques in ApoE or Ldlr single mutant mice. In ApoE,PDGFRβ Sm22D849V mice, the plaques consistently developed into fibroatheromas. Moreover, the aortic plaques exhibited neovascularization and intraplaque haemorrhage, which are common in advanced atherosclerotic lesions in humans. Neovascularization is thought to contribute to disease by providing a route for macrophages and other leucocytes to enter the plaques [33] . Intraplaque haemorrhage worsens atherosclerosis by depositing large amounts of free cholesterol from erythrocyte membranes [25] , [26] . In addition, iron deposits in atheromas may worsen atherosclerosis by increasing the formation of reactive oxygen species and oxidized LDL [34] . ApoE −/− mice do not typically develop coronary atherosclerosis without long-term (10 months) WD feeding [27] , [28] . ApoE −/− Akt1 −/− double mutants develop coronary atherosclerosis after 14 weeks of high cholesterol diet through mechanisms involving increased endothelial cell and macrophage apoptosis [35] . More dramatically, scavenger receptor B1 (SR-BI)-deficient mice on an ApoE −/− background develop severe coronary atherosclerosis by 5 weeks of age due to profound alterations in lipoprotein metabolism [36] . Thus, the PDGFRβ Sm22D849V mice combined with ApoE or Ldlr mutations provide a distinct model of atherosclerosis that may help define the role of VSMCs in plaque advancement and coronary heart disease. We provided genetic evidence that inflammation directly contributes to novel plaque formation in the thoracic aorta. Conditional deletion of STAT1 in ApoE +/+ VSMCs was sufficient to normalize much of the chemokine overexpression and inflammation caused by PDGF signalling. However, VSMC phenotype switching and adaptive remodelling (dilation) of the aorta persisted in STAT1 Sm22cKO PDGFRβ Sm22D849V double-mutant mice, indicating that these aspects of the phenotype are not dependent on STAT1. Even though aortic dilation persisted in double mutants, far fewer plaques occurred in the thoracic aorta. Thus, our data point to an inflammatory pathway as an important mechanism by which PDGF signalling amplifies atherosclerosis. We cannot completely exclude possible haemodynamic changes secondary to remodelling of the aorta as a contributing factor towards enhanced atherosclerosis, but our genetic evidence demonstrates that STAT1-linked inflammation is required. This inflammatory pathway involves PDGFRβ activation in VSMCs, activation of JAKs, tyrosine phosphorylation of STAT1, secretion of chemokines from VSMCs and accumulation of leucocytes in the adventitia and media of the aortic wall. Leukocyte accumulations were apparent in histological sections of PDGFRβ Sm22D849V adventitia ( Fig. 2d ). Intriguingly, recent studies highlight the potential of VSMCs to act as lymphoid tissue organizers by secreting chemokines (CXCL13, CCL21 and others) that promote lymphoid tissue neogenesis [37] , [38] . Furthermore, aged ApoE −/− mice develop tertiary lymphoid tissue in the aorta adventitia [39] . As we did not find well-organized lymphoid tissue in the adventitia, the relevance of these observations to our model is unknown. It is possible that our mice were too young at the time of analysis, or that the chemokines involved are not sufficient for the formation of organized lymphoid tissue. Specific chemokines we identified as STAT1-dependent PDGF targets have been previously shown to have pro-atherogenic functions. CCL2/MCP-1 and CCL5/RANTES are important chemoattractants for monocytes and macrophages in the atherosclerotic setting [40] , [41] , [42] , [43] . CXCL10/IP-10 modulates the balance of effector and regulatory T cells in atherosclerosis by activating the receptor CXCR3 (refs 44 , 45 ). There is evidence to suggest that the related chemokines CXCL9/MIG and CXCL11/ITAC also regulate T-cell trafficking in atherosclerosis [45] , [46] , [47] . Together, these data suggest that chemokines released by VSMCs work together to inflame the aorta, which may create new niches for plaque initiation when combined with hypercholesterolaemia. Arterial VSMCs have long been viewed as one of the major cell types involved in atherosclerosis [48] . Most recent work on plaque initiation has focused on the importance of inflammatory cells and endothelial cells, while VSMCs are more often discussed in the context of advanced atherosclerosis when VSMCs switch from a contractile to a secretory phenotype, proliferate, migrate into plaques and create fibrous cap structures. However, from human autopsy studies it is known that VSMCs predominate in the thickened arterial intima at atherosclerosis-prone sites even prior to the onset of plaque formation [49] , [50] , [51] . Therefore, it has been suggested that VSMCs might help initiate plaques at atherosclerosis-prone sites by transdifferentiating into foam cells [52] , [53] , by producing proteoglycans that trap lipoproteins [54] , by expressing adhesion molecules that recruit inflammatory cells [55] , or by enhancing the activity or survival of monocytes and macrophages [56] . Further investigation may reveal whether any of these disease processes are exacerbated in PDGFRβ Sm22D849V mice and whether they are modulated by the loss of STAT1. The D849V mutation in PDGFRβ increases basal and ligand-mediated signalling activity of PDGFRβ, which leads to constitutive phosphorylation of STAT1 in a JAK1/2-dependent manner. Phosphorylation of STAT1 in PDGF-treated cells was demonstrated over 20 years ago [57] , and our study now shows an in vivo role for the PDGFRβ–STAT1 signalling pathway in regulating the VSMC inflammatory phenotype. STAT1 knockout mice do not exhibit vascular phenotypes under basal conditions [58] , [59] . However, STAT1 may operate in VSMCs in a context-dependent manner, for instance during the response to injury and inflammation. STAT1 may be especially important under conditions where IFN-γ and PDGF are both present, as previous studies suggested interactions between the two signalling pathways [60] , [61] , [62] , [63] . Further work will be needed to understand the importance of VSMC-expressed STAT1 for atherosclerosis in standard ApoE - and Ldlr -deficient mice. This study shows that increased PDGFRβ signalling causes inflammation and VSMC dedifferentiation in vivo . In the setting of hypercholesterolaemia, PDGFRβ signalling promotes new plaque initiation at atherosclerosis-resistant sites and promotes the formation of fibroatheroma plaques with neovascularization and plaque rupture. A novel aspect of this study is the observation that initiation of plaques in the subendothelium of thoracic aorta requires inflammation of the adventitia and media. The conventional model of atherosclerosis has focused on the inner layers of the vessel, guided by the paradigm of endothelial cell activation, subendothelial inflammation, monocyte recruitment to the subendothelium and foam cell formation in the subendothelium. This view emphasizes inflammation beginning at the luminal side of the vessel wall and progressing outward, with the outer layers of the vessel playing a passive role. However, the present study contributes experimental evidence pointing towards the importance of outside-in mechanisms where inflammation of the adventitia and media creates new niches for atherosclerotic plaque initiation. Mice Sm22α-Cre;PDGFRβ +/D849V ( PDGFRβ Sm22D849V ) conditional knockin mice [18] were crossed to ApoE or Ldlr -deficient mice obtained from the Jackson Laboratory. STAT1 flox/flox mice were provided by L. Hennighausen (NIDDK, NIH, Bethesda, MD) [32] . Collagen1a1-EGFP transgenic reporter mice were provided by D. Brenner (UCSD, La Jolla, CA) [64] . All mice were maintained on a mixed C57BL/6;129 background and were fed standard chow or WD (diet#TD88137, Harlan Teklad). Some mice were injected with 15 mg kg −1 Crenolanib (Selleck Chemicals) for 5 consecutive days. Mutant mice were always compared with age and sex-matched controls that carried the appropriate Cre driver, and littermates were used whenever possible. We did not observe any vessel aneurism development (defined as focal dilation/weakening of the vessel wall), aortic dissection, kidney failure or tumour formation in any of the PDGFRβ Sm22D849V mutants we examined during the period of our study. All animal experiments were performed under approval from the Institutional Animal Care and Use Committee of the Oklahoma Medical Research Foundation. Isolation and culture of primary VSMCs Mouse VSMCs were isolated by the explant method from aortas of 6–8-weeks-old mice [65] . VSMCs were cultured in DMEM medium plus 10% FBS and antibiotics. All assays were performed at passages 2 to 5. To induce chemokine expression, wild-type VSMCs were serum starved in DMEM+0.5% FBS for 36 h, followed by stimulation with 10 ng ml −1 PDGF-BB (R&D Systems). For STAT phosphorylation experiments, 10 ng ml −1 mouse IFN-γ (EMD Millipore) served as a positive control. To block PDGFRβ activity, VSMCs were treated with 400 ng ml −1 Crenolanib for 2 h or 10 μM AG-1295 (Calbiochem) for 16 h. To block JAK1/JAK2 kinase activity, VSMCs were treated with 10 μM Rux for 16 h. STAT1 siRNA and nonsilencing control siRNA were obtained from Santa Cruz Biotechnology. Mouse VSMCs were transfected with siRNA for 48 h using Lipofectamine RNAiMAX (Invitrogen) according to the manufacturer’s instructions. RNA isolation and qRT–PCR Total RNA was extracted from cultured VSMCs using RNeasy Mini Kit (Qiagen). Reverse transcription to complementary DNA was performed using random primers and Superscript III RT (Invitrogen). Quantitative real-time PCR was performed using a Bio-Rad iCycler with iQ TM SYBR green master mix. Results were normalized relative to GAPDH unless indicated otherwise. Quantification of mouse chemokine proteins Mouse VSMCs were cultured in six-well plates. Chemokine protein levels in harvested conditioned media and mouse plasmas were determined using a multi-analyte ELISA kit (Qiagen MEM-009A) according to the manufacturer’s instructions. Aorta flow cytometry analysis Single-cell suspensions were prepared from the mouse aortas as described [20] . Briefly, mice were anaesthetized and perfused through the heart with PBS containing 10 U ml −1 heparin to remove blood from all vessels. After careful removal of the perivascular adipose tissue, the aortas were minced into small pieces and digested with 125 U ml −1 collagenase type XI, 60 U ml −1 hyaluronidase type I-s, 60 U ml −1 DNase1 and 450 U ml −1 collagenase type I (all enzymes were obtained from Sigma-Aldrich) in PBS containing 20 mM Hepes at 37 °C for 3 h. For separating adventitia and media, the aortas were predigested in enzyme cocktail (300 U ml −1 collagenase I and 10 U ml −1 Elastase in PBS) at 37 °C for 15 min and then the adventitia was carefully peeled away from the aorta. After filtering through a 70 μm filter, cells were resuspended in FACS buffer, and incubated with Fc-blocking antibody (eBioscience) for 15 min on ice before being stained with specific antibodies. Antibodies used were as follows: FITC-CD45.2, PE-CD11c, APC-CD3, APC-Cy7-CD19, PE-Cy7-NK1.1 and PerCy5.5-CD11b (all antibodies were obtained from Biolegend and used at 1:100 dilution). Cells were also stained with propidium iodide. After washing, immunofluorescence was detected by an LSR II (BD Biosciences). Data were analysed using FlowJo (Tree Star Inc.) software. Immunoprecipitation and western blotting VSMCs were lysed in RIPA buffer and protein contents were measured using the BCA assay (Sigma). Total lysates were immunoprecipitated with antibody against PDGFRβ (Santa Cruz Biotechnology, sc-432). Immunoprecipitates or cell lysates were subjected to western blotting with antibodies to phospho-STAT1 (Invitrogen 333400), phospho-STAT3 (Cell Signaling, 9145), phospho-STAT5 (Cell Signaling, 9359), β-Actin (Cell Signaling, 4970L), phosphotyrosine (Millipore, 05-321), total STAT1 (Millipore, 06-501), total PLCγ1 (Cell Signaling 2822) and phosphor-PLCγ1 (Cell Signaling 14008). Primary antibodies were used at 1:1,000. Horseradish peroxidase-conjugated secondary antibodies (Jackson ImmunoResearch) were used at 1:5,000. BrdU incorporation and labelling index Mice were injected with 50 mg kg −1 BrdU and then killed 24 h later. Aortas were perfused by cardiac puncture with PBS containing 10U ml −1 of heparin, and then with 4% paraformaldehyde (PFA), paraffin embedded and sectioned longitudinally. Cells were identified as VSMCs based on their position between the internal and external elastic lamina of the tunica media. Proliferating VSMCs (BrdU + ) were detected with anti-BrdU antibody (Sigma) at 1:20 dilution. Haematoxylin was used as a counterstain for nuclei. Blood pressure measurements Blood pressure was measured by the carotid catheter method. About 8–10-weeks-old mice were anaesthetized with a ketamine and xylazine mixture (70:6 mg kg −1 , intramuscular injection) and placed under warm light (37 °C). The left common carotid artery was carefully exposed via a 0.5- to 1.0-cm midline incision in the ventral neck region. The tip of the artery towards the head was ligated with a suture (5–0 silk), and the tip towards heart was occluded with a microclip (no. 18055–03; Fine Science Tool, Foster City, CA). A small cut was then made in the vessel wall using microscissors (no. 15000–08, Fine Science Tool). A catheter (PE10 tubing) containing a sterile 10% heparin–90% saline solution was inserted into the common carotid. Blood was directed to a pressure transducer through the catheter to obtain computerized blood pressure measurements (AD instruments) after removing the clip; (mean±s.e.m. n =6 mice per group). Serum lipid profiles Wild-type or PDGFRβ Sm22D849V mice from both sexes were fed chow diet for 2–3 months or WD for 24 weeks. ApoE and ApoE,PDGFRβ Sm22D849V mice were fed chow diet for 8–10 months or WD for 16 weeks. Blood was drawn from the facial vein with light anaesthesia and serum was separated by centrifugation. Cholesterol and triglyceride levels were determined by commercially available kits (BioVision and ThermoScientific) followed by spectrophotometric quantification. Qualitative analysis of tissues and atherosclerotic plaques For immunohistochemistry, aortas were perfused as above, and were post-fixed in 4% PFA overnight, then cryosectioned at 8 μm and stained with primary antibodies recognizing PECAM (BD Bioscience 553370, 1:100), αSMA (Sigma F3777, 1:250), MOMA-2 (AbD Serotec MCA519G, 1:100), F4/80 (Abcam ab6640, 1:100), SMMHC (Biomedical Technologies Inc. BT-562, 1:100) or Sm22α (Abcam ab10135, 1:100), with appropriate donkey secondary antibodies (Jackson ImmunoResearch). Immunofluorescence microscopy was performed with a Nikon Eclipse 80 i microscope connected to a digital camera. Final image processing was performed with Photoshop (Adobe). For histological stains, perfused aortas were post-fixed with Bouin’s solution, paraffin embedded and sectioned at 5 μm before staining with Movat’s pentachrome, Masson’s trichrome or Prussian blue. Formalin-fixed aortic roots were cryosectioned at 10 μm and stained with Oil red O. Quantitative analysis of plaques Mice were perfused as described above, followed by overnight post-fix with 4% PFA. For en face staining, the adventitia was thoroughly cleaned under dissecting microscope, and the aorta was cut open longitudinally and pinned on parafilm. Plaques were stained with Oil red O and photographed with a digital camera. For cross-sectional quantification of plaque progression, 5 μm serial paraffin sections from the indicated sites of the aorta were stained with haematoxylin and eosin. Plaques were imaged with a Nikon Eclipse 80 i microscope connected to a digital camera. Plaque area was then quantified with NIS.Elements D3.2 imaging software (Nikon Inc.) to obtain the maximum cross-sectional plaque area for each site. Fibrous cap thickness was quantified by choosing the largest necrotic core in a section and measuring the thinnest part of the fibrous cap. Representative images were finally processed with Photoshop (Adobe). Transmission electron microscopy Two-week-old mice were perfusion fixed through the heart, then thoracic aorta segments were isolated and immersion fixed with 1.5% glutaraldehyde and 2.5% PFA in 0.1 M HCl-Na cacodylate buffer for 2 h, then post-fixed for 90 min at 40 °C with 1% osmium tetraoxide in the same buffer and then incubated with 0.5% tannic acid for 30 min at room temperature. After dehydration in graded ethanol and propylene oxide treatment, specimens were embedded in epoxy resin. Sections were cut with a diamond knife, stained with lead citrate and uranyl acetate and examined with a Hitachi H-7600 electron microscope. Statistical analysis Data are expressed as mean±s.e.m. Statistical difference was analysed with the Student’s t -test. A value of P <0.05 was considered statistically significant. How to cite this article: He, C. et al . PDGFRβ signalling regulates local inflammation and synergizes with hypercholesterolaemia to promote atherosclerosis. Nat. Commun . 6:7770 doi: 10.1038/ncomms8770 (2015).